Termination chemistry-driven dislocation structure at SrTiO3/MgO heterointerfaces Exploiting the promise of nanocomposite oxides necessitates a detailed understanding of the dislocation structure at the interfaces, which governs diverse and technologically relevant properties. Here we report atomistic simulations demonstrating a strong dependence of the dislocation structure on the termination chemistry at the SrTiO 3 /MgO heterointerface. The SrO- and TiO 2 -terminated interfaces exhibit distinct nearest neighbour arrangements between cations and anions, leading to variations in local electrostatic interactions across the interface that ultimately dictate the dislocation structure. Networks of dislocations with different Burgers vectors and dislocation spacing characterize the two interfaces. These networks in turn influence the overall stability of and the behaviour of oxygen vacancies at the heterointerface, which will dictate vital properties such as mass transport at the interface. To date, the observed correlation between the dislocation structure and the termination chemistry at the interface has not been recognized, and offers novel avenues for fine-tuning oxide nanocomposites with enhanced functionalities. The last decade has witnessed unabated growth of research on oxide materials due to their wide-ranging applications that include information storage [1] , [2] , [3] , radiation-tolerant materials [4] , [5] , fuel cells [6] , [7] and batteries [8] . In the majority of these applications, vital properties of nanocomposite oxides are influenced or even controlled by oxide interfaces. Engineering nanocomposite oxides via precise control over the interfaces relies on fundamental understanding of the structure of those interfaces and their correlation with various properties. However, understanding the structure of these interfaces is complicated as oxide heterostructures can have significant mismatch between the two constituent phases wherein the atomic structure is strained or altered [9] , [10] , [11] , [12] , an outcome that has ramifications on the behaviour of defects and on the material properties. In addition, the influence of strain and misfit dislocations (MD) at oxide heterointerfaces on properties pertinent to energy applications is not well understood [13] . More importantly, as this information is not easily accessible experimentally due to buried interfaces and metastable heterostructures encountered during synthesis, theoretical frameworks providing insight into the structure and stability of nanocomposite oxides are valuable for designing next-generation oxide-based materials. In the present study, we use atomistic simulations to investigate the structure of model semicoherent SrTiO 3 (STO)/MgO interfaces in an attempt to understand the dislocation structure, and its influence on the overall behaviour of oxygen vacancies at the heterointerface. It is well established that dislocation structures at heterointerfaces depend on the orientation relationship due to strain between the two materials [9] , [10] , [14] , [15] , [16] . Here, for the same orientation relationship, we demonstrate strong dependence of dislocation structure at oxide heterointerfaces on the termination chemistry, wherein SrO- and TiO 2 -terminated STO/MgO interfaces exhibit notably different dislocation structures with varied dislocation spacing and Burgers vector. These differences are the consequence of local electrostatic interactions across the interface, which differ for the two terminations. The characteristic dislocation structures in turn impact the behaviour of oxygen vacancies at the interface, which would have repercussions on the transport properties at the interface and on radiation damage evolution of oxide nanocomposites. Such relationships between the structure and property in oxide heterointerfaces have not been established in the past, and offer the prospect of tuning the properties of oxide nanocomposites by varying the termination chemistry at the interface. Atomic-scale structure of the interface To predict atomic-scale structure of the interface, atomic models of STO/MgO interfaces were constructed with the experimentally observed [17] , [18] cube-on-cube orientation relationship where (001) STO ||(001) MgO ||interface and [010] STO ||[010] MgO . As lattice parameters are a STO =0.3905, nm and a MgO =0.4212, nm, the lattice mismatch arising from this orientation relationship is ~7.2%, indicating that 14 unit cells of STO must be matched to 13 unit cells of MgO to ensure a bicrystal with no extrinsic strain [17] (the misfit strain in this case is then 0.0012%). Minimizing misfit strain in the materials necessitates the formation of MDs at the interface. Maintaining the same geometrical parameters and cube-on-cube orientation relationship, two different interfaces were constructed, corresponding to SrO- and TiO 2 -terminated STO. The rationale behind such a scheme, which is consistent with experimental observations [17] , [18] , [19] , is that, while rocksalt MgO has one neutral (100) plane, the neutral perovskite STO (100) planes alternate between SrO and TiO 2 . The size of the supercell in the interface normal direction was ~4.3 nm. 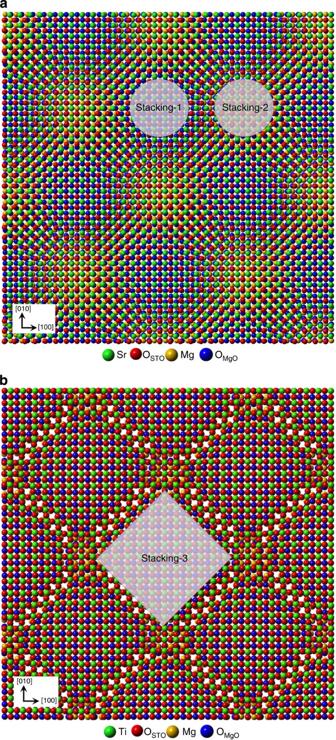Figure 1: Minimized STO/MgO interfaces. (a) SrO-terminated interface. (b) TiO2-terminated interface. OSTO(red) and OMgO(blue) are coloured differently for clarity. Cations in STO (Sr and Ti) are coloured green and gold corresponds to Mg. The view is normal (STO is above MgO in this view) to the interface plane. Only one atomic plane on each side of the interface is shown for clarity. Figure 1a,b presents views of the final minimized configurations of SrO- and TiO 2 -terminated interfaces, respectively, along the interfacial normal direction, providing a clear view of the dislocation structure at each interface. In the images shown in Fig. 1a,b , the relaxed supercells are extended in the x and y directions (2 × 2 × 1) for better visualization. These interfaces were found to be structurally stable on annealing at 2,000 K for 10 ps, wherein the SrO-terminated structure changed marginally. Henceforth, different regions of atomic arrangements will be correlated with different stackings and oxygen atoms will be denoted as O STO and O MgO depending on their respective location in STO and MgO. For the SrO-terminated interface, as indicated in Fig. 1a , there are two terraces (coherent regions) with different atomic stackings at the interface. The two stackings are stacking-1: O STO are over Mg and Sr are over Mg, while O MgO do not have nearest neighbours across the interface; stacking-2: Sr are over O MgO and O STO are over O MgO , whereas Mg do not have nearest neighbours across the interface. Thus, while both regions exhibit repulsive interactions, the nature of those repulsions is different (cation–cation for stacking-1 and anion–anion for stacking-2), and the two terraces are expected to have different chemical bonding and dissimilar energy. The intermediate region separating these terraces constitutes MD lines and MD intersections (MDIs). Figure 1: Minimized STO/MgO interfaces. ( a ) SrO-terminated interface. ( b ) TiO 2 -terminated interface. O STO (red) and O MgO (blue) are coloured differently for clarity. Cations in STO (Sr and Ti) are coloured green and gold corresponds to Mg. The view is normal (STO is above MgO in this view) to the interface plane. Only one atomic plane on each side of the interface is shown for clarity. Full size image As shown in Fig. 1b , for the TiO 2 -terminated interface, the principal stacking is stacking-3: Ti are over O MgO and O STO are over Mg, while additional O MgO in alternate columns do not have nearest neighbours across the interface. The intermediate region separating stacking-3 corresponds to MDs and MDIs, wherein Ti are over Mg and O STO are over O MgO and additional Mg in alternate columns do not have nearest neighbours across the interface. Evidently, in TiO 2 -terminated interface, stacking-3 has favourable electrostatic interactions, whereas MDIs will behave contrastingly due to repulsive interactions within a small region. A vital feature of these interfaces is that between the three possible stackings for SrO- and TiO 2 -terminated interfaces, only stacking-3, witnessed in the TiO 2 -terminated interface, involves an atomic arrangement with no repulsive nearest neighbours. In the remaining stackings, cation–cation or anion–anion nearest neighbours (or both) are present at the interface creating chemical frustration (unfavourable electrostatic interactions). On the basis of a similar electrostatic model, it was suggested that STO could not be grown on MgO unless the stacking sequence is initiated with TiO 2 planes [19] , although recent experiments have observed both interfaces [17] , [18] . The complex atomic arrangement at the STO/MgO interface within the coherent regions has been observed in the past, however, none of the studies consider different stackings in the same supercell, nor do they account for MDs at the interface due to system size limitations in first-principles calculations [20] , [21] , [22] . Disregistry analysis of dislocation structure at the interface To quantify the MD structures depicted in Fig. 1a,b , we performed disregistry analysis [23] , [24] across the interface plane for both SrO- and TiO 2 -terminated interfaces. For the disregistry analysis, the two interface layers nearest to the interface (one each from STO and MgO) were taken into account. To measure the disregistry, a reference state must be chosen in which the two adjoining neighbouring layers constituting the interface are coherent. To construct these coherent dichromatic pattern reference states [25] , we compressed the MgO layer and stretched the SrO layer (for the SrO-terminated interface) or the TiO 2 layer (in case of the TiO 2 -terminated interface) by equal amounts along the [100] and [010] directions. After constructing the reference states, a correspondence list of nearest neighbour atoms in the MgO and the STO side of the interface layers is compiled for each of the two reference configurations (that is, for the SrO- and TiO 2 -terminated interface models). Disregistry vectors are finally computed as where is the relative position between the i th and j th atom that form a pair in the reference and is the relative position between the same pair of atoms at the relaxed interface [23] , [24] . For the two interface models, we plot the components (screw) and (edge) of the disregistry vectors along directions and (parallel and normal to the set of MD lines, respectively) along the respective directions shown in Fig. 2a,b . Screw components in both cases are consistently close to zero, whereas the edge components in both the cases reveal step-like flat periodic regions that are formed as a result of the tendency of the interface to localize into terraces, while the steepest slope in between correspond to the dislocation cores that separate the terraces. Key parameters characterizing the two-dimensional (2D) dislocation network can be extracted from Fig. 2a,b . In each of the two cases, the difference between successive horizontal flat regions of the disregistry edge component is the magnitude of the net Burgers vector of the dislocation. On the other hand, the distance between successive horizontal regions along the abscissa provides spacing between the parallel sets of dislocations. Our analysis shows that for the SrO-terminated case, the MDs split into partials (with Burgers vector of ), while for the TiO 2 -terminated interface a full MD (with Burgers vector of ) is predicted. 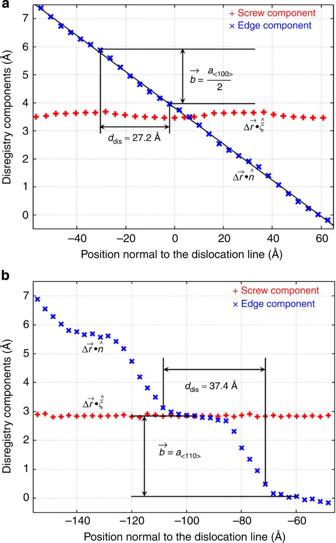Figure 2: Disregistry analysis of the STO/MgO interfaces. Disregistry components (edge and screw) as a function of disregistry positions for (a) SrO-terminated interface and (b) TiO2-terminated interface. The steps in the edge components of disregistry reveal the presence of interface dislocations. There is negligible screw character for dislocations in either interface. A black line is drawn inato show the changing slope. Figure 2: Disregistry analysis of the STO/MgO interfaces. Disregistry components (edge and screw) as a function of disregistry positions for ( a ) SrO-terminated interface and ( b ) TiO 2 -terminated interface. The steps in the edge components of disregistry reveal the presence of interface dislocations. There is negligible screw character for dislocations in either interface. A black line is drawn in a to show the changing slope. Full size image We verified our atomistic predictions to be consistent with the Frank–Bilby equation [26] , [27] , [28] , given as follows: For each interface, index k runs over all the unique sets of dislocation lines present at the interface, each with Burgers vector and separation length l k between the parallel lines within a given set. θ k denotes the angle between a dislocation line direction and the probe unit vector , measured in the anti-clockwise direction. D represents a deformation matrix that maps the coherent reference configuration on the natural structure. We find that for both SrO- and TiO 2 -terminated interfaces, our results obtained through disregistry analysis of our atomic structures are consistent with the Frank–Bilby equation. Generalized stacking energy of the interface The prediction of material stability and mechanical properties is critical for rational design of heterointerfaces. Stacking energy [29] , [30] , [31] is a critical parameter in the assessment of mechanical and structural properties of materials. The generalized stacking energy (GSE) of SrO- and TiO 2 -terminated interfaces has been calculated for the γ-surface projection [32] along <100> and <110> to assess the influence of the different chemical interactions in the different regions of the interface ( Fig. 1a,b ) on the total energy and stability of the system. GSEs were computed using [30] , [31] γ sf =( E S − E Ref )/ A , where E S and E Ref are the total potential energies of the sheared crystal at each displacement and the reference crystal, respectively, and A is the area of the interface plane. Compared with metals [29] , [30] , [31] , the choice of reference crystal ( E Ref ) is nontrivial for the STO/MgO interface as it involves two different terminations at the interface layer. For the SrO-terminated interface, the Sr–O MgO interaction is more repulsive than Mg–O STO . Accordingly, stacking-1 is energetically more favourable as compared with stacking-2. In the TiO 2 -terminated interface, there is only one stable stacking, stacking-3. Thus, stacking-1 and stacking-3 are taken as the reference structures for SrO- and TiO 2 -terminated interfaces, respectively. 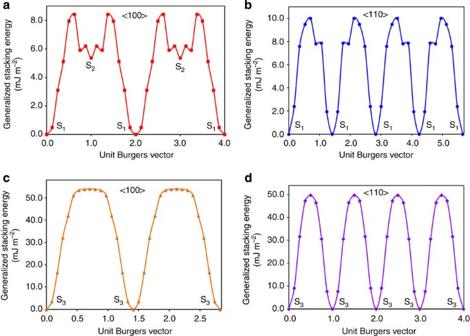Figure 3: GSEs of the STO/MgO interfaces. GSEs for SrO-terminated interface along (a) <100> and (b) <110> directions. GSEs for TiO2-terminated interface along (c) <100> and (d) <110> directions. S1, S2and S3correspond to stacking-1, stacking-2 and stacking-3, respectively. Figure 3 illustrates the curves generated from GSE calculations for γ-surface projections along <100> and <110> for both the SrO- and TiO 2 -terminated interfaces. In Fig. 3a for the SrO-terminated interface, two minima, one for stacking-1 and the other for stacking-2, characterize the curve along <100>. Conversely, along <110> ( Fig. 3b ), only one minimum is encountered corresponding to stacking-1. This behaviour can be correlated with the length of the Burgers vector b found from the disregistry analysis. For the SrO-terminated interface , starting with stacking-1, stacking-2 is encountered by moving along <100>, whereas stacking-1 is recovered by moving along <100> and along <110>. For the TiO 2 -terminated interface, a pattern qualitatively different to that observed for the SrO-terminated interface emerges, as curves along <100> ( Fig. 3c ) and <110> ( Fig. 3d ) are characterized by a single minima corresponding to stacking-3. For the TiO 2 -terminated interface , stacking-3 is recovered by moving along <100> and along <110>. In both cases, the maxima between the stable stackings correspond to structures associated with the MDs and MDIs. Further, the energy difference between individual stackings within each interface is very different. For instance, in the SrO-terminated interface, the energy difference between stacking-1 and MDI region is significantly lower (~10 mJ m −2 ) as compared with the energy difference between stacking-3 and MDI region observed in TiO 2 -terminated interface (~50 mJ m −2 ). Consequently, MDs in SrO-terminated interface will be more delocalized as compared with MDs in TiO 2 -terminated interface. Figure 3: GSEs of the STO/MgO interfaces. GSEs for SrO-terminated interface along ( a ) <100> and ( b ) <110> directions. GSEs for TiO 2 -terminated interface along ( c ) <100> and ( d ) <110> directions. S 1 , S 2 and S 3 correspond to stacking-1, stacking-2 and stacking-3, respectively. Full size image Work of adhesion of the interface The thermodynamic work of adhesion or adhesion energy ( W ad ), defined as the work done on the system to reversibly separate an interface into two free surfaces, is another quantity used for gauging the mechanical stability of the interface. Adhesion energies of SrO- and TiO 2 -terminated interfaces have been computed using [33] , [34] , [35] W ad ≡( E 1 + E 2 − E Int )/ A , where E 1 , E 2 and E Int are total energies of the isolated surface of slab 1, the isolated surface of slab 2 and the interface, respectively, and A is the total interface area. Contrary to first-principles-based computations, wherein the assumed coherency due to smaller cell sizes leads to errors in computing adhesion energies [36] , the present framework ensures a more realistic prediction due to the inclusion of MDs. Computed adhesion energies for SrO- and TiO 2 -terminated interfaces are 0.099 and 1.517 J m −2 respectively, suggesting that, while the latter is thermodynamically more stable, both are stable structures at 0 K. Of course, at finite temperature, we would expect a more complicated interfacial structure comprising all of the stackings with populations governed by Boltzmann statistics based on the respective energy differences and the formation of any boundaries between interfaces. The adhesion energies corroborate very well with the GSE calculations as well as reported theoretical results [20] , [21] , [22] , which indicate that for fully coherent models, the TiO 2 -terminated interface (stacking-3) is more stable due to the nature of bonding at the interface. In addition, some experiments indicate that epitaxial growth can be achieved only for TiO 2 -terminated interface, whereas SrO-terminated interface leads to islanding or surface roughening [19] . However, the adhesion energies also reveal that either SrO or TiO 2 truncation is possible, which is in very good agreement with recent experiments that reveal mixed terminations due to the presence of steps at the interface [17] , [18] . Nevertheless, this is contrary to theoretical calculations that report only TiO 2 -terminated interfaces as being thermodynamically stable [21] , [22] . Discrepancy between our results and previous theoretical calculations could be attributed to supercell size limitation in first-principles-based calculations, wherein MDs are not explicitly incorporated [20] , [21] , [22] , which may lead to errors in calculating adhesion energies [36] . Results for the adhesion energy emphasize the necessity for including MDs at semicoherent interfaces to accurately estimate the stability of oxide heterointerfaces. Oxygen vacancy energetics across the interface A final query is how the differing interfacial structures influence the behaviour of defects at the interfaces. To shed light on this behaviour, the relative energies of oxygen vacancies at the interface layers in SrO- and TiO 2 -terminated interfaces were computed. The rationale behind these computations is that oxygen vacancies, commonly encountered at oxide heterointerfaces during deposition [37] , [38] , strongly impact the structural, mechanical, transport and electrical properties of oxide nanocomposites. For the SrO-terminated interface, Fig. 4a,b displays maps of the relative oxygen vacancy energies at the interfacial STO and MgO layers, respectively. Oxygen vacancies strongly prefer to exist in the STO layer as compared with the MgO layer. Within the STO layer ( Fig. 4a ), oxygen vacancies strongly prefer stacking-2 as compared with stacking-1, MDIs and dislocation lines. Unlike the STO layer, due to higher oxygen density in the MgO layer ( Fig. 4b ), oxygen vacancies prefer both stacking-1 and stacking-2. Akin to STO layer, oxygen vacancies in the MgO layer evade MDIs and dislocation lines. Preference of oxygen vacancies to exist at the terraces can be attributed to the structure at the interface, wherein O STO are on top of O MgO (stacking-1) and O MgO do not have any nearest neighbour interaction across the interface (stacking-2), suggesting their removal is favourable. One remarkable outcome is that despite the O STO –O MgO nearest neighbour environment across the interface at stacking-2, oxygen removal is more favourable in the STO layer rather than being equally likely in both layers. This suggests that the Mg–O bond is much stronger than the O bonds in STO. Overall, at the SrO-terminated interface, vacancies exhibit a strong preference to reside in one of the terraces, but not in other regions of the interface. 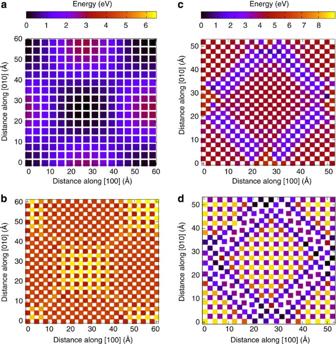Figure 4: Oxygen vacancy formation energies at the interfacial layers. (a) STO layer and (b) MgO layer in SrO-terminated interface. (c) STO layer and (d) MgO layer in TiO2-terminated interface. In all figures for individual layers, the view is normal to the interface plane. Energies are shifted so that 0 eV corresponds to most stable position for the oxygen vacancy within the respective interface. Figure 4: Oxygen vacancy formation energies at the interfacial layers. ( a ) STO layer and ( b ) MgO layer in SrO-terminated interface. ( c ) STO layer and ( d ) MgO layer in TiO 2 -terminated interface. In all figures for individual layers, the view is normal to the interface plane. Energies are shifted so that 0 eV corresponds to most stable position for the oxygen vacancy within the respective interface. Full size image Figure 4c,d shows maps of the relative oxygen vacancy energies at the interfacial STO and MgO layers, respectively, for the TiO 2 -terminated interface. In contrast to the SrO-terminated interface, oxygen vacancies prefer the MgO layer over the STO layer, although this preference is much weaker. As shown in Fig. 4c for the STO layer, oxygen vacancies prefer the dislocation lines and their immediate vicinity, whereas they avoid the terrace (stacking-3). Oxygen vacancies in the MgO layer ( Fig. 4d ) strongly favour MDIs and dislocations lines and their immediate neighbourhood. Preference of oxygen vacancies to exist at MDIs can be correlated with the structure at the interface, wherein O STO are on top of O MgO suggesting their removal is favourable. In contrast to the STO layer, the pattern observed in stacking-3 of the MgO layer varies with atomic column depending on the local atomic arrangement. Overall, at the TiO 2 -terminated interface, vacancies favour MDIs and dislocations lines, avoiding the terraces. It is critical to recognize that each data point corresponding to an oxygen vacancy energy depicted in Fig. 4 only emphasizes the most probable vacancy formation location at the interface independent of the existence of other defects in the material. Oxygen vacancies, typically positively charged in similar oxides [39] , [40] , lead to electrostatic interactions that alter the energetics of vacancies nearby. Furthermore, the formation of equilibrium space–charge regions [7] , [39] , [41] , [42] at the interface can lead to vacancy-rich dislocation cores and vacancy-depleted space–charge zones, which would further influence the oxygen vacancy energy and defect concentration. In addition, either oxygen-rich or oxygen-poor conditions [43] encountered during deposition would have a bearing on the oxygen vacancy energies. Overall, several competing effects dictate the oxygen vacancy energies and corresponding defect concentration across the interface. As a result, oxygen vacancy energies given in Fig. 4 are not adequate to accurately predict defect concentration profiles. Nonetheless, these energies ( Fig. 4 ) essentially reveal that the vacancy distribution and dynamics near different types of dislocations will be distinct, and thus demonstrate that the differences in interfacial structure we observe here will have important consequences for functionality. The present result suggesting that the oxygen vacancy is more favourable to exist in the MgO layer of TiO 2 -terminated interface is in disagreement with first-principles calculations [22] . The observed discrepancy can be attributed to the absence of MDIs in the first-principles calculations [21] , [22] and the presence of strain in coherent supercells, which can alter oxygen vacancy formation at oxide heterointerfaces [44] , [45] , [46] . For instance, using the present methodology for a coherent supercell of TiO 2 -terminated interface, we found that oxygen vacancy formation is more favourable in the STO layer in accord with reported first-principles calculations [22] , suggesting that the induced strain reverses the observed preference. A prominent attribute in both SrO- and TiO 2 -terminated interfaces is the strong variation in relative vacancy energy with the local atomic structure of the interface. This non-homogeneity in oxygen vacancy energies underpins the importance of understanding the dislocation structure at the interface. A single value for the oxygen vacancy formation energy at the interface, routinely extracted from first-principles calculations [22] , cannot elucidate this non-homogeneity. An intriguing disparity in the behaviour of oxygen vacancies at the two interfaces is their location preference, wherein they favour terraces in the SrO-terminated interface and MDIs and dislocation lines in the TiO 2 -terminated interface. The behaviour of oxygen vacancies observed in TiO 2 -terminated interface is similar to that of defects at metallic nanocomposites [15] , [16] , where MDIs are found to mitigate radiation damage by acting as sinks for radiation-induced point defects. Further, pipe diffusion along MDs is one potential mechanism found to be responsible for fast diffusion of vacancies in metallic heterointerfaces [47] . Our current results, although limited to oxygen vacancies, suggest that the TiO 2 -terminated interface would exhibit similar pipe diffusion mechanisms, which is responsible for radiation damage evolution in Y 2 O 3 (ref. 48 ). In addition, as oxide nanocomposites are increasingly used in solid oxide fuel cells and oxygen separation membranes [7] , the TiO 2 -terminated interface can serve as a model system for assessing the role of pipe diffusion for conductivity, as observed in yttria-stabilized zirconia [49] . In contrast, the SrO-terminated interface does not exhibit such behaviour, with vacancies concentrated in terraces separated by dislocations that act as barriers for migration. This suggests that properties such as ionic conductivity and defect annihilation will be significantly reduced at this interface as compared with the TiO 2 -terminated interface and the STO/MgO system serves as an ideal model to determine the role of MDs in ionic conductivity at interfaces. In summary, we have demonstrated that the dislocation structure in STO/MgO heterointerfaces is contingent on the termination chemistry at the interface, an outcome that dictates the interfacial stability and defect behaviour at the interface. Observed relationship between the termination chemistry and the dislocation structure of the interface has not been previously established, and offers potential avenues for improving transport properties and radiation damage resistance of oxide composites by controlling the termination layer at interfaces. In addition, the present findings also shed light on the complexity involved in accurately characterizing the structure of oxide heterointerfaces and emphasize the significance of understanding the MD structure as it influences vital properties of nanocomposites. Atomistic simulations Atomistic calculations with 3D periodic boundary conditions were performed within the framework of Large-scale Atomic/Molecular Massively Parallel Simulator (LAMMPS) [50] . Parameters for the Buckingham pair potential as derived by Busker et al. [51] were used for MgO and STO as they were fitted against the same O 2− —O 2− potential. For predicting dislocation structures, energy minimization was performed along all three supercell directions and the forces on all atoms were allowed to relax ( Fig. 1 ). GSEs have been computed using a supercell geometry, wherein coherent blocks of STO (SrO- and TiO 2 -terminated) and MgO are allowed to shear with respect to each other. For consistency, the same supercell size with periodic boundary conditions along x and y directions and free surface in the z direction was implemented for both the reference and sheared (faulted) interfaces [31] . Adhesion energy calculations were performed with supercells that include MDs. To ensure consistency and cancellation of errors in computing interface and surface energies, all adhesion energy calculations were performed using the same supercell dimensions for the respective interfaces [35] . For elucidating the oxygen vacancy behaviour across the interface, after the removal of each oxygen atom, energy minimization was performed wherein the atomic positions were allowed to fully relax before computing vacancy energies. Each oxygen vacancy has an associated formal charge of +2. For these computations, the atomic structure depicted in Fig. 1 was implemented. How to cite this article: Dholabhai, P. P. et al. Termination chemistry-driven dislocation structure at SrTiO 3 /MgO heterointerfaces. Nat. Commun. 5:5043 doi: 10.1038/ncomms6043 (2014).